Reproductive isolation related to mimetic divergence in the poison frogRanitomeya imitator In a mimetic radiation—when a single species evolves to resemble different model species—mimicry can drive within-species morphological diversification, and, potentially, speciation. While mimetic radiations have occurred in a variety of taxa, their role in speciation remains poorly understood. We study the Peruvian poison frog Ranitomeya imitator , a species that has undergone a mimetic radiation into four distinct morphs. Using a combination of colour–pattern analysis, landscape genetics and mate-choice experiments, we show that a mimetic shift in R. imitator is associated with a narrow phenotypic transition zone, neutral genetic divergence and assortative mating, suggesting that divergent selection to resemble different model species has led to a breakdown in gene flow between these two populations. These results extend the effects of mimicry on speciation into a vertebrate system and characterize an early stage of speciation where reproductive isolation between mimetic morphs is incomplete but evident. Elucidating the factors that promote population divergence and initiate speciation is key to understanding the evolution of biodiversity. Several studies have identified cases where divergent selection on ecologically relevant traits leads to partial or complete reproductive isolation or speciation [1] , [2] , [3] , [4] . Speciation is frequently studied by examining pairs of ‘good’ species and identifying current reproductive barriers [5] . However, these reproductive barriers may have arisen after speciation was complete, whereas other, currently incomplete barriers may have arisen earlier and been important during initial population divergence [6] . With the goal of investigating initial divergence, one can focus on the early stages of speciation, for example, populations of a single species showing incipient reproductive isolation. Mimicry can drive phenotypic convergence between distantly related species, but can also drive within-species diversification. This has led to impressive morphological radiations in diverse taxonomic groups such as catfish [7] , millipedes [8] , snakes [9] , bees [10] , frogs [11] , moths [12] and, most famously, Heliconius butterflies [13] . In Heliconius , selection for Müllerian mimicry (mimicry between unpalatable species) has led to intraspecific divergence in wing patterns, as different populations radiate into distinct mimicry rings [13] . These wing patterns are also used in mate choice, and morph-based assortative mating can arise as a byproduct of selection for wing mimicry [14] if accompanied by evolution of preferences. Studies of mimetic hybrid zones in Heliconius have yielded a range of examples highlighting the continuous nature of speciation. On one end of the continuum, hybrid zones can be narrow and characterized by strong assortative mating, neutral genetic divergence and infrequent hybridization [15] , [16] . On the other end of the continuum, hybrid zones can be wide, with little or no assortative mating, and with genetic divergence generally restricted to genomic regions controlling colour–pattern differences [17] . There are, however, few examples of ‘intermediate’ hybrid zones, where distinct mimetic morphs show intermediate levels of genetic divergence and/or premating isolation (but see ref. 18 ). By identifying cases where speciation appears to have started, but is not yet complete, we can better understand how freely interbreeding populations transition to reproductively isolated species. Neotropical poison frogs (Dendrobatidae) are diurnal, toxic frogs known for their striking warning colours. A number of species display remarkable intraspecific diversity in colour–pattern [19] , [20] , [21] , [22] , although in most cases the source of divergent selection among populations is unclear [23] , [24] , [25] , [26] , [27] . In Ranitomeya imitator , intraspecific divergence in colour–pattern is associated with selection for Müllerian mimicry [28] , which led to the establishment of four distinct mimetic morphs of this species in central Peru [29] . These morphs resemble three different model species (one of the model species, R. variabilis , has two morphs itself [21] , both mimicked by R. imitator ), and occur in different geographic regions, forming a ‘mosaic’ of mimetic morphs. Where different morphs come into contact, narrow hybrid (or ‘transition’) zones are formed [29] , similar to what has been observed in Heliconius butterflies. We have identified three such transition zones, making this study system useful for comparative analyses. Here we show that a mimetic shift in R. imitator is likely driving early-stage reproductive isolation among two of these mimetic morphs. We focus on the narrowest transition zone, which is found in the lowlands of north-central Peru and is formed between the ‘varadero’ morph, which mimics R. fantastica , and the ‘striped’ morph, which mimics the lowland morph of R. variabilis [30] ( Fig. 1 ; Supplementary Fig. 1 ). Our sampling along a transect crossing this transition zone reveals that there is a shift in several aspects of colour–pattern in R. imitator , including dorsal colour (yellow to orange), arm colour (pale greenish-blue to orange), leg colour (pale greenish-blue to navy blue) and dorsal pattern (uniform longitudinal stripes to colouration concentrated around the head). These shifts correspond to the colour–pattern of each model species ( Fig. 1 ; Supplementary Fig. 2 ), and are therefore likely involved in mimicry. Analyses of colour–pattern clines show that the transition zone is ~1–2 km wide and composed of phenotypic intermediates. Landscape genetic analyses indicate that neutral genetic divergence between morphs is primarily associated with divergence in mimetic colour–pattern, rather than geographic distance, suggesting that mimetic divergence has reduced gene flow between morphs. Using mate-choice experiments, we find evidence for assortative mating in one of the mimetic morphs, however, this mating preference is only present near the transition zone, consistent with reproductive character displacement (RCD). Taken together, these results suggest that mimetic divergence in R. imitator has led to a breakdown in gene flow between these two populations, potentially facilitated by assortative mating. 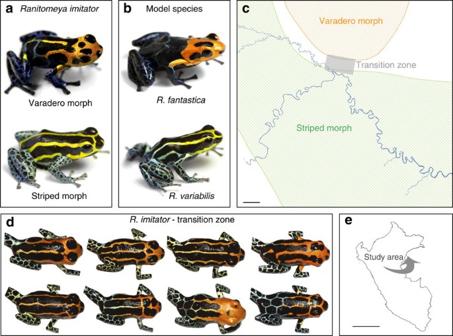Figure 1: Mimetic divergence inR. imitator. In central Peru, the mimic poison frogR. imitator(a) exhibits two mimetic morphs corresponding to two different model species (b). These morphs occupy distinct geographic areas (c), and form a narrow transition zone (grey box,c) characterized by phenotypic intermediates (d). Scale bar, 3 km (c). (e) Map of Peru showing study area (scale bar, 500 km). Figure 1: Mimetic divergence in R. imitator. In central Peru, the mimic poison frog R. imitator ( a ) exhibits two mimetic morphs corresponding to two different model species ( b ). These morphs occupy distinct geographic areas ( c ), and form a narrow transition zone (grey box, c ) characterized by phenotypic intermediates ( d ). Scale bar, 3 km ( c ). ( e ) Map of Peru showing study area (scale bar, 500 km). Full size image Colour–pattern clines Selection for different mimetic morphs across geographical areas should cause differentiation in mimetic traits. At the interface between distinct mimetic morphs, traits subject to divergent selection are expected to show a sigmoidal pattern of variation across this zone of mixing [31] . To quantify colour–pattern variation along the mimicry transect, we used a combination of spectrometry and computer-automated feature extraction to extract six colour–pattern variables in R. imitator . Transect variation in three of these colour–pattern variables (head colour, body colour and leg pattern) was best described by a linear model ( Fig. 2 ), suggesting gradual spatial change. However, due to our sampling pattern, we cannot rule out the possibility of a sigmoidal cline with a displaced centre for these colour–pattern variables. The remaining three colour–pattern variables (arm colour, leg colour and body pattern) were best described by a sigmoidal model ( Fig. 2 ), suggesting that these aspects of the colour–pattern are under divergent selection. If multiple aspects of the colour–pattern are involved in mimetic resemblance, then shifts in traits should coincide geographically. We tested for cline coincidence among arm colour, leg colour and body pattern by comparing Akaike weights ( w i ) between two models: one where cline centre is constrained to a single parameter shared across all three data sets and one where centre is unshared. A common centre was found for all three colour–pattern variables without a significant reduction in model fit ( w i shared centre model=0.841; w i unshared centre model=0.159), indicating coincidence among the three colour–pattern clines. The point estimate for the shared centre parameter was 0.54 km (that is, 0.54 km N from the a priori -estimated centre), corresponding to 1.25 km N from the village of Varadero ( Supplementary Fig. 1 ). An alternative explanation for coincident clines is recent secondary contact between divergent populations (see below for discussion of primary versus secondary contact). 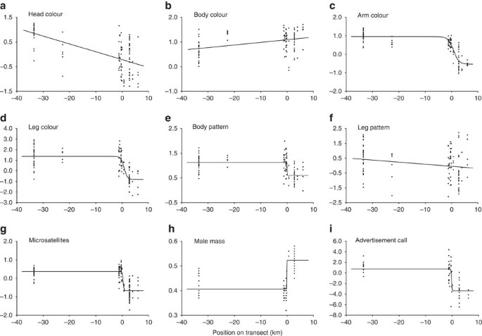Figure 2: Clines in colour–pattern, microsatellites, male mass and advertisement calls. In all panels, trait values for individualR. imitator(represented by dots) are plotted along the geographic transect (xaxis). (a–f) Colour–pattern variation (yaxis: kernel discriminant score; values closer to +1 indicate closer similarity toR. variabilisand closer to −1R. fantastica); (g) microsatellite variation (yaxis: first major axis from factorial correspondence analysis (FCA)); (h) male mass (yaxis: grams); and (i) advertisement call variation (yaxis: linear discriminant score). The fit line for each variable represents the best-supported model describing transect variation and parameter point estimates. Figure 2: Clines in colour–pattern, microsatellites, male mass and advertisement calls. In all panels, trait values for individual R. imitator (represented by dots) are plotted along the geographic transect ( x axis). ( a – f ) Colour–pattern variation ( y axis: kernel discriminant score; values closer to +1 indicate closer similarity to R. variabilis and closer to −1 R. fantastica ); ( g ) microsatellite variation ( y axis: first major axis from factorial correspondence analysis (FCA)); ( h ) male mass ( y axis: grams); and ( i ) advertisement call variation ( y axis: linear discriminant score). The fit line for each variable represents the best-supported model describing transect variation and parameter point estimates. Full size image In a tension zone model [31] , where divergent selection is opposed by dispersal, the width of the cline reflects a balance of selection (which narrows a cline) and dispersal (which widens a cline). Differences in cline widths among different traits may be due to differences in the strength of selection on loci underlying those traits. If different traits are controlled by the same number of loci, those under stronger selection should show narrower clines than those under weaker selection. We tested for a common cline width (concordance) among all six colour–pattern variables. A common width could not be found among all six variables without a reduction in model fit ( w i shared width model=0.273; w i unshared width model=0.727), indicating that some colour–pattern variables show non-concordant widths. This was due to the inclusion of the three non-sigmoidal variables, as it was possible to fit a common width of 2.27 km among the three variables showing a sigmoidal pattern of variation ( w i shared width model=0.747; w i unshared width model=0.253). Cline width should be primarily a function of selection strength (assuming constant dispersal), so the evidence that these three clines can be constrained to a common width suggests equivalent strength of selection on arm colour, leg colour and body pattern. This could also suggest a common genetic basis or linkage among all three traits, although colour and pattern elements in dendrobatids are likely controlled by different genes [32] . Landscape genetics Reduced gene flow between adaptively diverged populations (isolation by adaptation; IBA) is a key prediction of ecological speciation [1] . This results in a positive correlation between adaptive ecological divergence and genetic differentiation among populations after controlling for the effect of isolation by distance (IBD) [33] . Results from the Structure analysis ( Fig. 3a ) indicate the presence of three genetic groups within the study area. One of these groups ( Fig. 3b ) is associated with an allopatric population, while two of the groups ( Fig. 3c,d ) form a sharp break at the mimetic transition zone. These latter two groups still show some evidence of genetic exchange, as there were a few individuals with a striped colour–pattern but a varadero genotype, and vice-versa ( Fig. 3 ). The narrow genetic cline is also characterized by a peak in linkage disequilibrium ( Supplementary Fig. 3 ), further suggesting a barrier to gene flow among the two mimetic morphs. The coincidence of genetic clines and colour–pattern clines was supported by a factorial correspondence analysis, where the cline centre on the first major axis (0.31 km) is almost identical to the shared colour–pattern cline centre (0.54 km), supporting the hypothesis that a shift in mimicry has led to a breakdown in gene flow among mimetic morphs. Using a causal modelling framework, the best-supported hypothesis was one where colour–pattern distance (IBA), but not geographic distance (IBD), was correlated with genetic distance among populations. Multiple-matrix regression [34] yielded similar results, except that both colour–pattern distance ( r 2 =0.427, P =0.006) and geographic distance ( r 2 =0.230, P =0.001) were accounted as significant predictors of genetic distance. However, the correlation coefficient for colour–pattern distance is nearly twice that of geographic distance, indicating that IBA is a stronger determinant of among-population genetic divergence than is IBD. An alternative interpretation for these results is mimetic divergence in allopatry followed by secondary contact. This could explain the neutral genetic divergence among these two populations, however, one would expect the microsatellite cline to be wider than the observed 0.54 km unless contact happened very recently (see below). 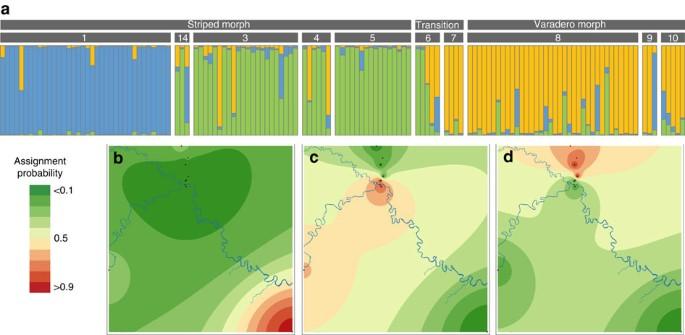Figure 3: Genetic structure between mimetic morphs ofR. imitator. (a) We used the software Structure 2.3.4 to analyse the multilocus microsatellite data set and assign individuals ofR. imitatorto each ofKpopulations. The optimal number of inferred populations wasK=3 (shown). Vertical bars indicate membership fractions to inferred groups 1 (blue), 2 (green), and 3 (orange). Horizontal grey bars represent the morph (upper bar) and sampling localities (lower bar). (b–d) Spatial genetic structure of each of the three genetic groups as inferred by Structure. We projected the Structure output to a map by interpolating the average probability assignment score of each population to each inferred group using inverse-distance-weighted interpolation in ArcGIS. (b) Probability assignment to group 1, (c) probability assignment to group 2 and (d) probability assignment to group 3. Figure 3: Genetic structure between mimetic morphs of R. imitator. ( a ) We used the software Structure 2.3.4 to analyse the multilocus microsatellite data set and assign individuals of R. imitator to each of K populations. The optimal number of inferred populations was K= 3 (shown). Vertical bars indicate membership fractions to inferred groups 1 (blue), 2 (green), and 3 (orange). Horizontal grey bars represent the morph (upper bar) and sampling localities (lower bar). ( b – d ) Spatial genetic structure of each of the three genetic groups as inferred by Structure. We projected the Structure output to a map by interpolating the average probability assignment score of each population to each inferred group using inverse-distance-weighted interpolation in ArcGIS. ( b ) Probability assignment to group 1, ( c ) probability assignment to group 2 and ( d ) probability assignment to group 3. Full size image Mate-choice experiments One potential mechanism for a breakdown of gene flow between adaptively diverged populations is morph-based assortative mating [35] . To address the role of assortative mating, we conducted triad mate-choice experiments in which we introduced two females (one of each morphs) into the terrarium of a given male, and measured the amount of courtship time between the male and female. This is equivalent to a mutual choice test, which is appropriate here as R. imitator is monogamous [36] , and therefore both sexes should be choosy. We tested preferences in three populations: striped allopatric, striped transition and varadero, allowing us to address two questions (1) whether courtship preferences differ between the striped-transition and varadero populations, and (2) whether courtship preferences differ among the two populations of the striped morph. Using generalized linear mixed models (GLMM), we found an overall significant effect of male origin ( χ 2 1,55 =16.518, P =0.00026), indicating that mate preferences were significantly different across populations. A post hoc test revealed that the preferences in the striped-allopatric and varadero populations were not significantly different ( χ 2 1,22 =3.096, false discovery rate (FDR)-adjusted P =0.078), with neither population showing a significant preference ( Fig. 4 ). However, preferences between the striped-transition and varadero populations were significantly different ( χ 2 1,33 =11.986, FDR-adjusted P =0.00161), mainly due to the striped-transition population’s preference towards its own morph ( Fig. 4 ), which indicates that mating preferences have diverged between these two populations across the transition zone. Finally, preferences between the striped-allopatric and striped-transition populations were significantly different ( χ 2 1,29 =9.748, FDR-adjusted P =0.00269), suggesting that mating preferences in the striped-transition population are stronger at the mimetic transition zone. 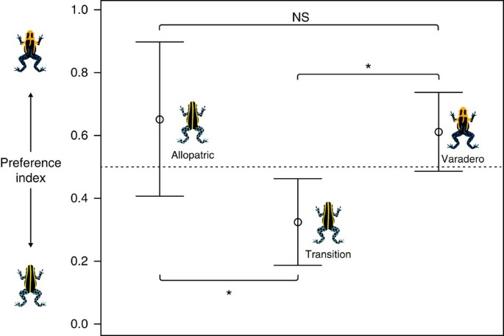Figure 4: Courtship preferences inR. imitator. For display on the figure, raw courtship times for each trial were converted to a ‘preference index’, which was calculated by dividing the time a male spent courting the varadero female by the time spent courting the varadero female+time spent courting the striped female (that is, dividing by total courtship time). This index therefore ranges from 0 (all courtship with striped female) to 1 (all courtship with varadero female), with a value of 0.5 (indicated by the dotted line) indicating no preference. Open circles show the mean preference index for each population; error bars represent 95% confidence intervals. Icons next to the error bars represent the morph of the male used in the experiment. Asterisks indicate significant differences from the GLMM (P<0.05) from thepost hoctests, following FDR adjustment for multiple comparisons. Sample sizes are as follows: striped allopatric,N=10; striped transition,N=19; varadero,N=26. Figure 4: Courtship preferences in R. imitator . For display on the figure, raw courtship times for each trial were converted to a ‘preference index’, which was calculated by dividing the time a male spent courting the varadero female by the time spent courting the varadero female+time spent courting the striped female (that is, dividing by total courtship time). This index therefore ranges from 0 (all courtship with striped female) to 1 (all courtship with varadero female), with a value of 0.5 (indicated by the dotted line) indicating no preference. Open circles show the mean preference index for each population; error bars represent 95% confidence intervals. Icons next to the error bars represent the morph of the male used in the experiment. Asterisks indicate significant differences from the GLMM ( P <0.05) from the post hoc tests, following FDR adjustment for multiple comparisons. Sample sizes are as follows: striped allopatric, N= 10; striped transition, N= 19; varadero, N= 26. Full size image Bioacoustics During our sampling, there were apparent differences in the advertisement calls of the striped and varadero morphs, which could represent a potential premating isolating mechanism between the two morphs. To determine whether the pattern of call variation coincided with the mimetic transition zone, we recorded the calls of R. imitator across the sampling transect. The call of R. imitator is a short, musical trill of 0.44–1.07 s, with trills (or ‘notes’) repeated roughly every 4–20 s, and a dominant frequency of 4,710–5,660 Hz. Each note is composed of 16–32 pulses, with an average pulse rate of 24–30 pulses per second [21] . Note length was negatively correlated with temperature ( r 2 =0.115, P =0.006), and pulse rate was positively correlated with temperature ( r 2 =0.259, P <0.001). To account for this, we standardized each of the three bioacoustic variables by calculating regression residuals against temperature. After temperature standardization, two bioacoustic variables showed a sigmoidal rather than linear pattern of variation across the transect (note length: Akaike weight ( w i ) linear model=0.032, w i sigmoidal model=0.967; dominant frequency: w i linear model=0.006; w i sigmoidal model=0.992). The point estimates of cline centre were similar (note length centre=−0.14 km; dominant frequency centre=−0.41 km), indicating that the shift in these two call parameters occurs in roughly the same geographic location. Furthermore, the estimated cline centres both occur very close to the estimated colour–pattern and microsatellite cline centres (within <1 km), indicating that the shift in call characteristics occurs in the same place as the shift in colour–pattern and microsatellites. For pulse rate, the linear model was favoured ( w i linear model=0.830, w i sigmoidal model=0.138), indicating a smooth, rather than abrupt, transition across the putative transition zone. To derive a single metric-describing call variation, we used a linear discriminant analysis to derive a discriminant score where the two groups for classification were defined as the populations on the end points of the transect (that is, populations 1 and 10 in Supplementary Table 1 ). Both note length and dominant frequency contributed substantially to the discriminant function, whereas pulse rate did not (standardized canonical discriminant function coefficients: dominant frequency=1.343; note length=−1.189; pulse rate=0.162). This metric showed a sigmoidal pattern of variation with similar cline centre and width as observed in the colour–pattern metrics ( Fig. 2 ; Supplementary Table 2 ). Our mate-choice trials found that the preferences in the two striped populations we studied were stronger in the striped-transition zone population relative to the striped-allopatric population, a pattern consistent with RCD. However, our experimental design is limited in terms of inferring RCD given that we only tested three populations, and therefore, assuming that mating preferences vary among populations, there is a one in three chance that the strongest preference will be in striped-transition population. A much more robust test of RCD would involve testing multiple populations to determine whether contact among morphs explains variation in mating preferences. Patterns of enhanced mating preferences in areas of contact have, however, been observed in mimetic Heliconius butterflies. For example, H. melpomene populations that are sympatric with H. cydno display stronger mating preferences relative to allopatric populations [37] . In another example, mating preferences in both H. cydno and H. pachinus are much stronger in sympatry than allopatry [38] . One explanation for this pattern is reinforcement, where mate preferences are strengthened in zones of sympatry to avoid producing unfit hybrids. However, several other processes can result in a pattern of enhanced mate preferences in zones of sympatry (for example, differential fusion hypothesis and ‘noisy neighbour’ hypothesis; see ref. 6 for review). In this case, as non-mimetic hybrids may suffer fitness costs if they experience higher predation rates [39] , adaptations to avoid cross-morph matings are expected to be favoured by selection. In addition to a shift in colour–pattern and microsatellites at the transition zone, we found a shift in body mass and certain aspects of the advertisement call. Striped frogs south of the transition zone tend to have a smaller body size and a shorter, more highly pitched call compared with the varadero morph north of the transition zone. For both body size and advertisement calls, variation along the transect is best described by a sigmoidal cline with centres coinciding with the colour–pattern and genetic clines ( Supplementary Table 4 ), further supporting the existence of a transition zone. This also supports the possibility for secondary contact, where clines are expected to be congruent for multiple traits. One possible explanation for the shift in body size is that R. variabilis , the model species of the smaller, striped morph of R. imitator , is smaller than R. fantastica , the model species of the varadero morph ( R. variabilis mass: , n =3; R. fantastica mass: , n =4). Thus, size could represent a mimetic adaptation. As our experiments did not address the specific cue used in mate choice, the roles of colour–pattern, body size and advertisement calls in mediating mate choice in this system should be investigated further. As we have mentioned above, secondary contact among differentially adapted populations could give rise to many of the observed cline patterns. One plausible scenario here would be mimetic divergence in allopatry, followed by secondary contact. Determining whether hybrid zones are the result of primary or secondary contact without historical evidence is difficult [31] . However, secondary contact with neutral diffusion is unlikely given our dispersal estimate in R. imitator of 0.095 km per generation (see Supplementary Methods for details on dispersal calculations). The cline created by secondary contact with subsequent neutral diffusion would exceed the observed overall cline width (0.97 km, see Supplementary Table 4 , model D) in only 17 generations, or ~11 years. Considering secondary contact, a more likely scenario is that the cline is maintained by some isolating barrier. In either case (primary or secondary contact), the cline is associated with a shift in mimicry, and may be maintained, at least in part, by assortative mating. Overall, the existence of a narrow cline, as well as moderate genetic divergence between morphs ( F ST between mimetic morphs is 0.065–0.077), suggests that mimetic divergence may be playing a key role driving early-stage speciation in a vertebrate system. Data availability Colour–pattern data, advertisement call data, mate-choice data and the full microsatellite data set are available at Dryad (doi:10.5061/dryad.rd586) . Sample collection and transect description For colour–pattern analyses, we sampled a total of 127 R. imitator from 15 localities in the department of Loreto, Peru. Ten of these localities (localities 1–10 in Fig. 1 ) lie on a rough north-south transect 40 km in length, running from the village of Micaela Bastidas in the south to 7 km N from the village of San Gabriel de Varadero in the north. We sampled an additional five localities off the transect but still relevant for inferring the spatial arrangement of the two focal morphs of R. imitator . For genetic analyses, we sampled 136 R. imitator from 10 localities. Tissue samples for genetic analysis (toe clips) were taken with sterile surgical scissors and preserved in 96% ethanol before extraction. In most cases, both tissue samples and colour–pattern measurements were taken from each frog, although there were some localities where only genetic data were collected or only colour–pattern data were collected (see Supplementary Table 1 for details). In addition, we took colour–pattern measurements from the two putative model species: 7 R. variabilis from Pongo de Cainarachi (representative of the typical lowland R. variabilis morph) and 7 R. fantastica collected from San Gabriel de Varadero. Because the transect is not perfectly linear, we calculated transect position as straight-line distance from the putative transition zone centre, with localities south of this point given a negative sign and localities north of this point given a positive sign. The initial centre point (latitude/longitude: −5.70653°, −76.41427°) used in these calculations was estimated from field observations where an apparent shift in colour–pattern occurred. Therefore, instances where the estimated cline centre from nonlinear regression was close to zero indicate a close fit to our field observations. Cline centre estimates with a negative sign indicate the inferred cline centre to be south of the initial centre point, whereas positive values indicate the cline centre to be north of the initial centre point. Colour and pattern quantification To quantify frog colour, we measured the spectral reflectance at specific points on the dorsal surfaces of the mimic species ( R. imitator ) and both model species ( R. variabilis and R. fantastica ). Two measurements were taken on the head (right and left sides), four on the body (right and left sides of mid-body and rump) and two on the legs (dorsal surface of right and left thighs). Reflectance measurements were taken using an Ocean Optics USB4000 spectrometer with an LS-1 tungsten–halogen light source and Ocean Optics SpectraSuite software. A black plastic tip was used on the end of the probe so that measurements were always taken at a distance of 3 mm from the skin and at a 45° angle. White standards were measured for every other frog using an Ocean Optics WS-1-SL white reflectance standard to account for lamp drift. Spectral data were then processed in Avicol version 6 software [40] using Endler’s segment model [41] calculated between 450–700 nm. This model calculates brightness (Qt), chroma (C), hue (H) and two Euclidean coordinates representing position in a two-dimensional colour space: blue-yellow axis position (MS) and red-green axis position (LM). Measurements within body regions (head, body and legs) were averaged. In addition to the spectrometer measurements, we measured upper-arm colouration using the colour-picker tool (set to a 5 × 5 pixel average) in Adobe Photoshop CS4 on dorsal photos of each frog, recording the average intensities of red, green and blue channels on two points on each upper arm. Photos were taken on a white background using a Canon Rebel XS DSLR with a Canon EF 100 mm macro lens and the camera flash. We quantified frog pattern by a collection of local image descriptors. The descriptors were automatically extracted from images of every individual and collected in a feature matrix. Three types of descriptors were extracted: a colour/non-colour ratio, gradient-orientation histograms and shape-index histograms [42] , [43] , [44] . Collectively, these capture zeroth-, first- and second-order image structure. A spatial pooling scheme was used to separately collect information at four interest points: left leg, right leg, lower and upper back. At each of these interest points, pattern variation occurs on a distinct scale, wherefore the descriptors were extracted according to a scale-space formulation [45] . Colour/non-colour ratios were extracted for every interest point on a single scale; gradient-orientation histograms for every interest point on two different scales and two orientation bins (horizontal and vertical), and shape-index histograms were only extracted for the legs on two scales in five bins equidistantly spaced between − π /2 and π /2. This summed up to a total of 4 · (1+2 · 2+2 · 5)=60 features per individual. To reduce the multivariate colour and pattern data to a single descriptive metric per body region, we used kernel discriminant analysis [46] , where the two model species ( R. variabilis and R. fantastica ) represented the training groups used for classification. This procedure assigns a discriminant score to each R. imitator individual on the basis of their similarity to either model species, and thus can be thought of as a ‘mimicry score’. The analysis can be constrained to include only subsets of the variables to derive a metric for different body regions, for example, leg colour variation in R. imitator . Kernel-based analysis is implicitly capable of estimating nonlinear effects, making it more suitable for non-normally distributed features, such as the colour metrics output from Avicol. Using this procedure, we derived colour metrics for four body regions (head, body, legs and arm) and pattern metrics for two body regions (dorsum and legs). For additional details on kernel discriminant analysis, see Supplementary Methods , Supplementary Table 5 , and Supplementary Figs 4 and 5 . Cline analysis To describe clinal variation in colour–pattern elements (as well as average male mass, advertisement call and microsatellites; see Supplementary Methods ), and in particular to estimate cline width, we performed nonlinear regression using a four-parameter sigmoid tanh function where c is the centre of the cline, w is the cline width and y max and y min are the maximum and minimum trait values (that is, the trait values at the tails of the cline). This uses the cline model of Szymura and Barton (ref. 47 ), except that the minimum and maximum trait values are free to take on any value. Parameter searches were done using the solver function in Excel using a least-squares optimality criterion. Solver was run using the generalized reduced gradient (GRG) nonlinear algorithm with the following settings: convergence=0.0001; central derivatives; multistart on; population size=100. To evaluate whether the data were adequately described by a ‘flat’ model (constant trait value across the transect) or a linear model (smooth transition), we fit these models, in addition to the sigmoid model, as candidate models. A flat model consists of a single parameter (population mean) defined as the grand mean of all individuals and is invariant across the transect. A linear model has two parameters, slope and y intercept, and was fit with linear regression. To evaluate which of the three models (one-parameter flat, two-parameter linear or four-parameter sigmoid) was a better fit to the data, we calculated ΔAICc and Akaike weights ( w i ) for each model (methods following ref. 48 ) using the residual sum of squares divided by the sample size as the likelihood criterion. Confidence intervals on parameter estimates were calculated using a Monte Carlo resampling method using the software GraphPad Prism. Briefly, this procedure involves the following steps: first, data are simulated for each observed x value using best-fit parameters of the observed cline, with scatter added by drawing data points randomly from a hypothetical normally distributed population with a s.d. equal to the observed S y . x (s.d. of the residuals). A cline is then fit to the simulated data and best-fit values of each parameter are recorded. This process is then repeated for a number of iterations, each time generating a new simulated data set, fitting a cline to that data set and recording parameter estimates. By using observed x values (that is, actual sampling locations) and observed residual variation, we are essentially simulating the distribution of cline parameter estimates that we might observe if we resampled the entire transect multiple times. Simulations were run for 10,000 generations and 95% confidence intervals were calculated on the simulation parameter estimates. We tested for common centre (coincidence) and common width (concordance) among clines using global nonlinear regression. This method compares model fit when certain parameters are shared versus unshared among different variables. Under a scenario where all variables shift at the same position on the transect, a common centre parameter can be fit across all measured variables without a substantial reduction in model fit. This is expected, for example, in a scenario where there is a shift in the selective regime for one mimetic colour–pattern in one area versus another area along the transect. If the width of a cline on a phenotypic trait is a function of the strength of selection on that trait, a global width parameter may be expected when selection acts at similar strength on all traits; however, if selection is strong on some traits and weak on others, this will cause different cline widths and thus a common width parameter will not adequately fit all the data. A common width may also be expected when linkage disequilibrium is high in the centre of the hybrid zone, as is observed here ( Supplementary Fig. 3 ). We evaluated four models representing different combinations of shared and unshared parameters ( Supplementary Table 4 ): (a) no constraint (each variable with unique centre and width), (b) centres constrained to be equal, width unconstrained, (c) width constrained to be equal, centres unconstrained, and (d) centre constrained to be equal and width constrained to be equal. Best-fit shared parameter searches were done by fitting shared parameters to all data sets simultaneously, while unshared parameters were free to take on unique values for each data set. Goodness of fit was assessed by calculating ΔAICc for each model. Mate-choice experimental design and analysis To test for morph-based mating preferences, we conducted triad mate-choice experiments in which we introduced two females (one of each morph) into the terrarium of a given male for 1 h, and measured the amount of courtship time between the male and the varadero female versus the male and the striped female. For details on the populations we sampled, as well as details on husbandry and experimental protocols, see Supplementary Methods . In R. imitator , courtship is usually initiated when a calling male approaches a female. The female may then either reciprocate by following the male to a suitable oviposition site while the male continues calling, or show no interest [49] . The conditions of our mate-choice experiments allowed these behaviours to take place in that a male was free to initiate courtship with either female, and the female was free to reciprocate interest or not. Male initiation of courtship is readily observable in captivity as males (a) initiate a courtship call (shorter and more rapid than an advertisement call) and/or (b) begin to move in a staccato-like walk, often moving their rear legs erratically. Thus, when a male engaged in either of these behaviours in the vicinity of a female, this marked the initiation of courtship. Courtship was deemed to have ended under the following conditions: (a) the male, having initiated courtship, moves away and the female does not pursue or (b) the female moves away and the male does not pursue. A trial was excluded when one or both females remained hidden in the gravel during the trial, thus precluding any possibility for choice. Using these criteria, we measured in each trial the total amount of courtship between the male and the varadero female versus the male and the striped female. Typically, in this kind of experimental setup, the two females to be introduced to the male would be matched for mass to control for any confounding effects of mass on preference. However, in this case, matching for mass was not feasible because the varadero population is larger than either striped population (striped-allopatric females , s.d.=0.05 g, n =43; striped-transition females , s.d.=0.04 g, n =18; varadero females , s.d.=0.05 g, n =30), severely limiting the number of potential female combinations (for example, only the four heaviest striped-transition females would have qualified to be matched with the six smallest varadero females). To control for differences between females, we used a paired-samples’ experimental design whereby a given pair of females was presented to a male of each morph. This design therefore addresses the question of how changing male morph type alters courtship probabilities when female identity is held constant. To analyse mate-choice data, we used GLMM using the glmmADMB package [50] in R version 3.0.2 (ref. 51 ) with an underlying beta-binomial error distribution to test whether the time males spent courting each female morph was influenced by male population origin. ‘Pair ID’ (that is, a unique identifier assigned to each female pair) was used as a random effect to account for the paired-samples’ experimental design. Following a significant result of the overall GLMM, we conducted post hoc tests to determine: (1) whether courtship preferences differ among morphs (specifically, comparing striped allopatric with varadero, and striped transition with varadero) and (2) whether courtship preferences differ among populations of the same morph (comparing striped allopatric to striped transition). Post hoc tests were run using the same GLMM procedure described above, except that we restricted the analysis to the populations of interest. To account for multiple comparisons, we adjusted P values using a FDR protocol [52] accounting for the fact that we conducted three post hoc tests. The protocols we used were approved by East Carolina University’s Institutional Animal Care and Use Committee (AUP permit #D225a) before the start of this study. Landscape genetics We used a causal modelling framework [33] , [53] to test specific hypotheses of how geographic distance and colour–pattern differentiation between populations are associated with genetic distance. In landscape genetics, causal modelling uses Mantel tests and partial Mantel tests to evaluate alternative models explaining genetic distance between populations. Each model carries a set of statistical predictions; the model with all its predictions upheld is the one with the strongest support. In an IBD scenario, a significant correlation is expected between a geographic distance matrix (independent variable set) and a genetic distance matrix (dependent variable set). By using partial Mantel tests, the correlation between two dissimilarity matrices can be quantified while controlling for the effect of a third covariant matrix. For example, a partial Mantel test between colour–pattern distance and genetic distance with geographic distance as covariant matrix tests for the correlation between colour–pattern distance and genetic distance after the effects of geographic distance are removed. We used one measure of geographic distance (Euclidean distance), one measure of genetic distance (Nei’s D ) and one measure of colour–pattern distance (difference in discriminant score, see below) to test three models of genetic isolation. Details on each model and their associated predictions are given in Supplementary Table 3 . Causal modelling is often used to test how various landscape factors influence genetic isolation among populations [53] , [54] . This can be useful for species occupying heterogeneous habitats, where straight-line distance between populations may not be the most likely corridor of gene flow. However, in our case, all populations of R. imitator are from a contiguous lowland rainforest habitat without any geographic barriers separating populations. The only two substantial barriers in this area, the Huallaga River and the Cordillera Escalera Mountains, are located to the east and south, respectively, of all sampling sites. Therefore, for the geographic distance matrix, we simply calculated pairwise straight-line distance between populations. For the genetic distance matrix, we calculated Nei’s genetic distance ( D ′) between all pairs of populations in GenAlEx version 6.5 (ref. 55 ). To generate a colour–pattern distance matrix, we calculated pairwise differences in discriminant score from the kernel discriminant function analysis. Thus, because this analysis takes into account features of the model species, it can be thought of as a composite difference in mimetic colour–pattern. In addition to causal modelling, we used a multiple-matrix regression method [34] to quantify the relative effects of geographic distance and colour–pattern distance on genetic distance. This method is similar to Mantel and partial Mantel tests but incorporates multiple regressions, such that the relative effects of two or more predictor variables on genetic distance can be quantified, as can the overall fit of the model. Multiple-matrix regression was run with 10,000 permutations using the R script provided in ref. 34 . For details on microsatellite-genotyping protocols, Structure analyses and factorial correspondence analyses, see Supplementary Methods and Supplementary Table 6 . Bioacoustics We recorded the advertisement calls of 58 R. imitator from eight localities. These localities are all located on the colour–pattern/microsatellite transect spanning the transition zone and thus can be used for cline analysis. Calls were recorded on a Marantz PMD660 solid state recorder using a Sennheiser ME 66-K6 microphone and analysed in Raven Pro version 1.3 (ref. 56 ). We quantified advertisement calls by measuring the following parameters: note length (measured from the start of the first pulse to the end of the last pulse), pulse rate (defined as pulse count divided by note time) and dominant frequency (the frequency at which peak amplitude is registered). For each male, a recording generally consisted of several notes. Measurements were always taken on at least three notes and then averaged for each male. As temperature is known to have a strong influence on certain aspects of amphibian calls [19] , we took temperature measurements alongside each call recording in the same microhabitat as the calling male, which we then used to standardize call parameters by calculating regression residuals against temperature. We fit clines to each call parameter separately, plus a ‘composite’ call score that we calculated using a linear discriminant analysis. How to cite this article : Twomey, E. et al. Reproductive isolation related to mimetic divergence in the poison frog Ranitomeya imitator . Nat. Commun . 5:4749 doi: 10.1038/5749 (2014).